Surface reconstruction and chemical evolution of stoichiometric layered cathode materials for lithium-ion batteries The present study sheds light on the long-standing challenges associated with high-voltage operation of LiNi x Mn x Co 1−2x O 2 cathode materials for lithium-ion batteries. Using correlated ensemble-averaged high-throughput X-ray absorption spectroscopy and spatially resolved electron microscopy and spectroscopy, here we report structural reconstruction (formation of a surface reduced layer, to transition) and chemical evolution (formation of a surface reaction layer) at the surface of LiNi x Mn x Co 1−2x O 2 particles. These are primarily responsible for the prevailing capacity fading and impedance buildup under high-voltage cycling conditions, as well as the first-cycle coulombic inefficiency. It was found that the surface reconstruction exhibits a strong anisotropic characteristic, which predominantly occurs along lithium diffusion channels. Furthermore, the surface reaction layer is composed of lithium fluoride embedded in a complex organic matrix. This work sets a refined example for the study of surface reconstruction and chemical evolution in battery materials using combined diagnostic tools at complementary length scales. Chemical evolution and structural transformations at the surface of a material directly influence characteristics relevant to a wide range of prominent applications including heterogeneous catalysis [1] , [2] , [3] and energy storage [4] , [5] . Structural and/or chemical rearrangements at surfaces determine the way a material interacts with its surrounding environment, thus controlling the functionalities of the material [6] , [7] , [8] , [9] , [10] . Specifically, the surfaces of lithium-ion battery electrodes evolve simultaneously with charge–discharge cycling (that is, in situ surface reconstruction and formation of a surface reaction layer (SRL)) that can lead to deterioration of performance [4] , [5] , [11] . An improved understanding of in situ surface reconstruction phenomena imparts knowledge not only for understanding degradation mechanisms for battery electrodes but also to provide insights into the surface functionalization for enhanced cyclability [12] , [13] . The investigation of in situ surface reconstruction of layered cathode materials, such as stoichiometric LiNi x Mn x Co 1−2x O 2 (that is, NMC), lithium-rich Li(Li y Ni x−y Mn x Co 1−2x )O 2 , lithium-rich/manganese-rich (composite layered–layered) xLi 2 MnO 3 ·(1−x)LiMO 2 (M=Mn, Ni, Co, and so on) materials, is technologically significant as they represent a group of materials with the potential to improve energy densities and reduce costs for plug-in hybrid electric vehicles and electric vehicles [14] , [15] , [16] , [17] . Practical implementation of some of these materials is thwarted by their high first-cycle coulombic inefficiencies [17] , [18] , [19] , [20] , capacity fading [18] , [21] and voltage instability [20] , [21] , [22] , especially during high-voltage operation. Specifically, high-voltage charge capacities achieved in lithium-rich/manganese-rich layered cathodes are directly associated with various irreversible electrochemical processes including oxygen loss and concomitant lithium ion removal [23] and electrode/electrolyte reactions [24] . With respect to regular NMC materials, although improved high-voltage cyclability (2.0–4.7 V versus Li + /Li) was recently achieved when a small percentage of Co was substituted with Ti (<4%), capacity fading still occurred after extended charge–discharge cycles [18] . Due to the structural and chemical complexities of these layered structures, their fading mechanisms have not been fully resolved. Electron microscopy studies indicated that, in lithium and manganese-rich materials, the capacity fading and voltage decay were partially attributed to structural reconstruction inducing a transition from the layered structure to spinel and/or rock-salt structures at the surface and/or in the bulk [5] , [17] , [25] , [26] . A recent study investigated the atomic structure of Li 2 MnO 3 after partial delithiation and re-lithiation to enable improved understanding of lithium-rich/manganese-rich materials [27] . However, these studies were mainly performed using spatially resolved techniques, thereby inevitably lacking relevance to large-scale battery electrodes and failing to account for the inhomogeneous nature of battery electrodes [28] , [29] , [30] . In addition, the role of electrode–electrolyte interactions in the surface reconstruction and chemical evolution has been rarely studied. The elucidation of the surface reconstruction of stoichiometric NMC materials should provide insights into the fading mechanisms not only for these compounds but also complement the mechanistic paradigm for more complex layered structures including lithium-rich and manganese-rich materials. In order to achieve a statistically viable and spatially visible elucidation (in real space) for surface phenomena on electrode materials, diagnostic techniques with complementary length scales should be implemented, including high-throughput synchrotron X-ray absorption spectroscopy (XAS) and atomic-scale scanning transmission electron microscopy (STEM) and electron energy loss spectroscopy (EELS). Here, we report the surface reconstruction and chemical evolution of stoichiometric NMC layered structures, using ensemble-averaged synchrotron XAS coupled with atomic-scale STEM-EELS, where the surface reconstruction and chemical evolution refer to the formations of surface reduced layer ( to transition) and SRL, respectively. Our results reveal that the surface reconstruction occurs simultaneously with charge–discharge cycles and is strongly determined by the upper voltage limits used during cycling, electrolyte exposure and crystal orientations. Furthermore, the major lithium-containing phase in the SRL is identified as lithium fluoride (LiF) embedded in a complex amorphous organic matrix. The present study provides insights into the surface reconstruction and chemical evolution in NMC materials and directly illustrates the origin(s) of the long-standing challenges involved in cycling NMC materials to high voltages, such as capacity fading, impedance increases and first-cycle coulombic inefficiency. Finally, the study complements the mechanistic understanding of the surface reconstruction in layered materials and sheds light on the possible advantages of conformal functionalization on the surfaces of NMC particles. Characterization of pristine materials LiNi 0.4 Mn 0.4 Co 0.18 Ti 0.02 O 2 (abbreviated NMC hereafter) powders with different particle size distributions were used for this study, because previous studies have shown that partial Ti substitution in NMCs results in higher practical specific capacities, better capacity retention upon cycling to 4.7 V versus Li + /Li, and decreased first-cycle coulombic inefficiencies compared with baseline electrodes [18] , [19] . The ratio of transition metals was verified to be close to stoichiometric LiNi 0.4 Mn 0.4 Co 0.18 Ti 0.02 O 2 ( Supplementary Fig. 1 ). Extensive analysis was performed on the pristine materials to verify the homogeneity of the surface and bulk prior to electrochemical implementation. The combinatorial evaluation was done using a variety of X-ray and electron-based techniques and is shown in Fig. 1 . The irregularly shaped primary particles of the NMC powder ranged in size from ~100–250 nm across ( Fig. 1a ), indicating that the surface is terminated with various crystal orientations. 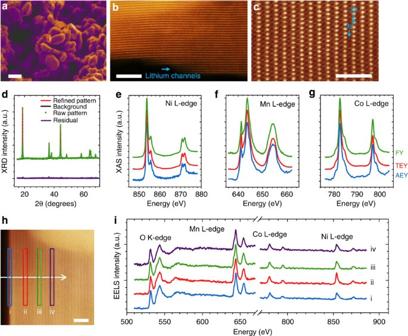Figure 1: Crystal structure and electronic structure of pristine NMC materials. (a) SEM image. (b) High-resolution Z-contrast ADF-STEM image. (c) Atomic resolution Z-contrast ADF-STEM image along the [100] zone axis, with the3aand3bsites indicated in the image. (d) XRD pattern with Rietveld refinement (fitted parameters are given inSupplementary Table 1). XAS spectra of (e) Ni L-edge, (f) Mn L-edge and (g) Co L-edge using AEY (blue), TEY (red) and FY (green) modes. (h,i) EELS spectra integrated from areas (i), (ii), (iii) and (iv); see alsoSupplementary Fig. 3for the spectroscopic imaging of the pristine surface. The scale bars ina,b,candhare 200 nm, 5 nm, 2 nm and 5 nm, respectively. Figure 1: Crystal structure and electronic structure of pristine NMC materials. ( a ) SEM image. ( b ) High-resolution Z-contrast ADF-STEM image. ( c ) Atomic resolution Z-contrast ADF-STEM image along the [100] zone axis, with the 3a and 3b sites indicated in the image. ( d ) XRD pattern with Rietveld refinement (fitted parameters are given in Supplementary Table 1 ). XAS spectra of ( e ) Ni L-edge, ( f ) Mn L-edge and ( g ) Co L-edge using AEY (blue), TEY (red) and FY (green) modes. ( h , i ) EELS spectra integrated from areas (i), (ii), (iii) and (iv); see also Supplementary Fig. 3 for the spectroscopic imaging of the pristine surface. The scale bars in a , b , c and h are 200 nm, 5 nm, 2 nm and 5 nm, respectively. Full size image The specific surface area of the material was measured to be 9 m g −2 by N 2 physisorption using the Brunauer–Emmett–Teller method ( Supplementary Fig. 2 ). An extensive number of atomic resolution annular dark-field STEM (ADF-STEM) images were obtained and representative ones are shown in Fig. 1b,c . STEM-EELS analysis was performed for the particle shown in Fig. 1b , and it was found that the transition metal oxidation state remains constant from the surface to the bulk ( Supplementary Fig. 3 ). Because ADF-STEM images approximately reflect the Z-contrast of materials, the images demonstrate that the material exhibits a well-defined layered structure, and the position of transition metals ( 3b sites) are atomically resolved along the [100] zone axis ( Fig. 1c ). Note that lithium ( 3a sites) and oxygen ( 6c sites) are not visible in the Z-contrast ADF-STEM image due to their low atomic masses. Powder X-ray diffraction (XRD) confirmed that the NMC has the expected layered structure ( Fig. 1d ). The refined lattice parameters are consistent with those reported previously for this composition [18] and are summarized in Supplementary Table 1 . Depth profiling of the electronic structure was carried out using XAS and STEM-EELS. Transition metal L-edge XAS and EELS measure the dipole allowed transitions from metal 2 p orbitals to unoccupied metal 3 d orbitals [31] , [32] , [33] and indirectly probe the local hybridization states for metal-oxygen octahedral units [34] in an NMC material. Transition metal L-edge XAS is superior to K-edge XAS in terms of resolving local hybridization states, as the former directly probes the unoccupied 3 d states in the metal 3 d -oxygen 2 p hybridized octahedral crystal field. Furthermore, L-edge XAS allows different sample depths to be probed from surface to bulk, depending on the detection modes. In the configuration used for this study, Auger electron yield (AEY), total electron yield (TEY) and fluorescence yield (FY) yield information about the chemical environments with depth sensitivities of 1–2 nm, 2–5 nm and 50 nm, respectively. Note that the FY probing depth is smaller than the particle size of the NMC materials, thus the signal primarily originates from the NMC particles on the top layer of the electrode rather than in the bulk of the composite electrode (typical thickness ~ 76 μm, Supplementary Fig. 4 ). XAS L-edge spectra of the transition metals exhibit almost identical shapes (for example, Ni3p 3/2 and Ni3p 1/2 splitting features) and L2,3 normalized intensities in AEY, TEY and FY modes ( Fig. 1e–g ), which suggest an ensemble-averaged chemical homogeneity in the NMC material. Finally, the formal oxidation states of Ni, Mn and Co are determined to be +2, +4 and +3, respectively, as expected [31] , [35] , [36] , [37] . Furthermore, the formal oxidation state of Ti is +4, and the shape of L-edge verifies the Ti substitution in the layered lattice ( Supplementary Fig. 5 ). A series of EELS area integrated spectra was recorded to directly assess the homogeneity of the chemical environment in a single NMC particle ( Fig. 1h ) and representative ones are displayed in Fig. 1i . The corresponding transition metal L-edge spectra exhibit no variation in the shapes or L3/L2 ratios at different probing positions. Furthermore, the O K-edge shows identical pre-edge peaks that are associated with the transitions from O 1 s to O 2 p -metal 3 d hybridized states and are sensitive to the oxidation states of transition metals [38] , [39] , which implies that the average oxidation states of transition metals remain constant from the top surfaces to volumes deep in the bulk. The above ensemble-averaged and spatially resolved spectroscopic studies allow us to conclude that the pristine NMC material exhibits a well-defined crystal structure with a homogenous distribution of the electronic structure. Furthermore, the homogeneity is not affected by the NMC particle size ( Supplementary Fig. 6 ). Such comprehensive investigation of homogeneity is rarely reported in the literature, although its establishment is critical for resolving the effects of electrochemistry on surface reconstruction and chemical evolution. Electrochemical tests of NMC materials The electrochemical performances of the NMC materials were evaluated in lithium half-cells, and the cycled electrodes were collected for the subsequent synchrotron X-ray and electron spectroscopy based investigation. There are distinct differences in behaviour between the high-voltage cycling (2.0–4.7 V) and lower-voltage cycling (2.0–4.3 V). The NMC material shows a gradually sloping charge profile with no evidence of the high-voltage plateau associated with irreversible loss of lithium and oxygen, commonly seen during electrochemical oxidation of lithium-excess compounds under these conditions [16] , [22] . Nevertheless, when repeatedly charged to 4.7 V versus Li + /Li, the capacity of the NMC electrode decreased with each cycle, while it fades very little during cycling between 2.0–4.3 V ( Fig. 2a–c ). Furthermore, the potential hysteresis between lithium deintercalation (charging) and intercalation (discharging) increased gradually during high-voltage cycling (indicated by the arrows in Fig. 2a ); namely, larger overpotentials were observed for both processes. Because cycling was carried out between set voltage limits, this impedance rise also contributed to the apparent capacity fading. In contrast, capacity retention was much better when using a lower-voltage limit on charge, that is, when cycling between 2.0–4.3 V ( Fig. 2b,c ). Such pronounced dependence on the voltage cutoff is partially caused by increased cell impedance under the high-voltage cycling conditions, as shown in Fig. 2d . The Nyquist plots of the impedance data are composed of a semicircle at high frequencies and Warburg tails at low frequencies, which correspond to charge transfer resistance and mass transfer resistance, respectively. Both charge transfer resistance and mass transfer resistance markedly increased after the extended high-voltage cycling indicated by the increased semicircle radius and the decreased slope of Warburg tail ( Fig. 2d ). In contrast, the charge transfer resistance slightly decreased after lower-voltage cycling between 2.0–4.3 V ( Fig. 2d ), which is likely attributed to cell conditioning and minimal surface reconstruction between 2.0–4.3 V (discussed below). An impedance rise was also observed when the NMC electrode was exposed to the electrolytic solution for an extended period ( Fig. 2e ) without being cycled. The similarities in the behaviour suggest that the NMC electrodes undergo similar modifications under conditions of cycling and electrolytic solution exposure, although to a lesser degree for the latter. 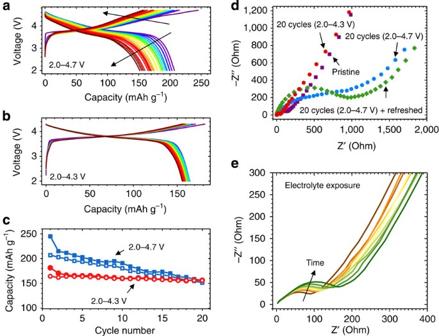Figure 2: Battery cycling performance of NMC materials. (a) Charge–discharge profiles at 2.0–4.7 V for 20 cycles at C/20, where the arrows indicate the gradual capacity fading and potential hysteresis. (b) Charge–discharge profiles at 2.0–4.3 V for 20 cycles at C/20. (c) Charge and discharge capacities as functions of cycle number at 2.0–4.7 V (blue square) and 2.0–4.3 V (red circle), respectively. The solid and open data points represent charge and discharge capacities, respectively. (d) Nyquist plots of impedance data obtained on cells containing electrodes in the pristine state, cycled at 2.0–4.3 V for 20 cycles, cycled at 2.0–4.7 V for 20 cycles and in the refreshed state (that is, rinsed with DMC, reassembled with fresh electrolyte after 20 cycles at 2.0–4.7 V). (e) A series of Nyquist plots for a pristine NMC electrode exposed to electrolytic solution for various periods up to 7 days. The exposure durations were 0 h (pristine), 5 h, 10 h, 1 day, 2 days, 3 days, 4 days, 5 days and 7 days. Figure 2: Battery cycling performance of NMC materials. ( a ) Charge–discharge profiles at 2.0–4.7 V for 20 cycles at C/20, where the arrows indicate the gradual capacity fading and potential hysteresis. ( b ) Charge–discharge profiles at 2.0–4.3 V for 20 cycles at C/20. ( c ) Charge and discharge capacities as functions of cycle number at 2.0–4.7 V (blue square) and 2.0–4.3 V (red circle), respectively. The solid and open data points represent charge and discharge capacities, respectively. ( d ) Nyquist plots of impedance data obtained on cells containing electrodes in the pristine state, cycled at 2.0–4.3 V for 20 cycles, cycled at 2.0–4.7 V for 20 cycles and in the refreshed state (that is, rinsed with DMC, reassembled with fresh electrolyte after 20 cycles at 2.0–4.7 V). ( e ) A series of Nyquist plots for a pristine NMC electrode exposed to electrolytic solution for various periods up to 7 days. The exposure durations were 0 h (pristine), 5 h, 10 h, 1 day, 2 days, 3 days, 4 days, 5 days and 7 days. Full size image Post analysis of NMC materials A correlated study using XAS, EELS and STEM imaging was performed to elucidate the mechanism of capacity fading and impedance rise in NMC cathodes under high-voltage cycling conditions. XAS/TEY is suitable for probing electronic structures at the top few nanometres due to the limited penetration depth of soft X-rays [40] . Because the measurements were performed on electrodes in the fully discharged state, nickel consistently showed a formal oxidation state of +2 after extended charge–discharge cycles ( Supplementary Fig. 7 ). In contrast, manganese and cobalt underwent significant changes upon cycling. The contribution from the low-energy shoulders of Mn L3- and Co L3-edges grew gradually with increasing numbers of cycles ( Fig. 3a,b ), indicating an evolution of transition metal 3 d bands to higher occupancies, that is, reduced oxidation states [35] , [36] , [41] . Furthermore, the oxidation states of transition metals exhibited depth-dependent characteristics, as shown by the direct comparison of AEY, TEY and FY spectra in Fig. 3c,d . The low-energy components of Mn L-edge and Co L-edge spectra were more obvious in the AEY mode than those in the TEY and FY modes. Therefore, the reduced Mn and Co species are primarily located at the surface. However, the high-energy component of the L3-edge was always present even in the surface-sensitive AEY mode, which suggests that the reduced Mn and Co species were not evenly distributed on individual NMC particles at the surfaces of the NMC electrodes. This observation coincides with previous studies that show that the charge distribution on the electrode surfaces is inhomogeneous in nature [30] . It is plausible that the reduced species were dominant on certain facets of individual NMC crystals, and that some surfaces exposed to incident X-rays retained the pristine electronic structure. Our subsequent investigation by ADF-STEM imaging further supports this hypothesis. An EELS line scanning profile was obtained on a particle cycled five times ( Fig. 3e–h ). The variation of the Mn oxidation state along the scanning direction is evident by the blue shift of the absolute energy onset and the reduced L3/L2 ratio [33] . A calculation based on the linear combination of Mn 2+ and Mn 4+ was performed and the corresponding concentration profiles are presented in Fig. 3h . The concentrations of Mn 2+ and Mn 4+ were inversely correlated along the scanning direction, with Mn 2+ primarily dominant on the surface. The thickness of the surface reduced layer was 2 nm for this particle, determined by using the intersections of Mn 2+ and Mn 4+ concentration profiles ( Fig. 3h ). An equivalent experimental protocol was applied to an NMC particle cycled 20 times. Along the identical crystal orientation, the thickness of the surface reduced layer increased to ~3.4 nm ( Supplementary Fig. 8 ). However, low-voltage cycling (2.0–4.3 V) yielded a surface reduced layer with a thickness of 2 nm after 20 cycles ( Supplementary Fig. 9 ). Another NMC material with identical composition yet smaller particle size was studied to probe the effect of particle size on the surface reduced layer, and the results show that the particle size imposes negligible effects on surface reduced layer within the range in this study ( Supplementary Fig. 10 ), and had similar cycling behaviour ( Supplementary Fig. 11 ). 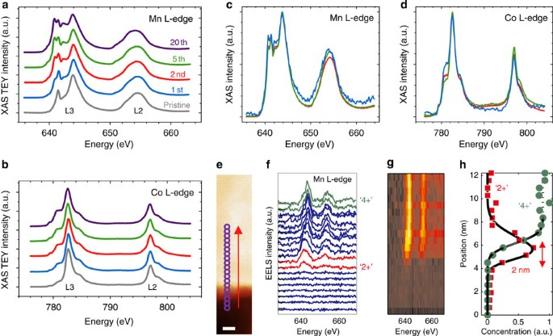Figure 3: Surface reconstruction and chemical evolution. (a) Mn L-edge XAS/TEY spectra and (b) Co L-edge XAS/TEY spectra after the designated number of cycles. (c) Mn L-edge XAS spectra and (d) Co L-edge XAS spectra for an electrode after two charge–discharge cycles in the AEY (blue), TEY (red) and FY (green) modes. EELS line scan profile for an NMC particle along the001direction after five cycles: (e) STEM image for the scanning pathway, (f) Mn L-edge EELS spectra along the scanning pathway, (g) 2D EELS map visualizing the peak shift and (h) concentration profiles for Mn2+and Mn4+obtained from the data using a linear combination method. All the measurements were performed on electrodes in the fully discharged state after cycled between 2–4.7 V versus Li+/Li. The scale bar in (e) is 2 nm. Figure 3: Surface reconstruction and chemical evolution. ( a ) Mn L-edge XAS/TEY spectra and ( b ) Co L-edge XAS/TEY spectra after the designated number of cycles. ( c ) Mn L-edge XAS spectra and ( d ) Co L-edge XAS spectra for an electrode after two charge–discharge cycles in the AEY (blue), TEY (red) and FY (green) modes. EELS line scan profile for an NMC particle along the 001 direction after five cycles: ( e ) STEM image for the scanning pathway, ( f ) Mn L-edge EELS spectra along the scanning pathway, ( g ) 2D EELS map visualizing the peak shift and ( h ) concentration profiles for Mn 2+ and Mn 4+ obtained from the data using a linear combination method. All the measurements were performed on electrodes in the fully discharged state after cycled between 2–4.7 V versus Li + /Li. The scale bar in ( e ) is 2 nm. Full size image In addition to the surface reduced layer on the active NMC materials, a surface reaction layer (SRL) was observed after extended charge–discharge cycles ( Supplementary Fig. 12 ). EELS revealed that the SRL consisted of a LiF phase in a complex organic matrix ( Supplementary Fig. 12 ). The SRL buildup is partially responsible for the impedance rise ( Fig. 2d ). The emergence of the SRL is mainly attributed to the repeated high-voltage electrochemical processes, because it was barely observed in the electrode that was cycled to the low voltage ( Supplementary Fig. 13 ) or exposed to the LiPF 6 /EC-DMC solution for 7 days, without being cycled ( Supplementary Fig. 14 ). The capacity retention of NMC materials is compromised when high-voltage cycling, such as 4.7 V versus Li/Li + , is used. Here we show that the surface reduced layer is related to the inferior capacity retention observed under high-voltage cycling conditions. As shown in Fig. 4a,b , the relative amounts of reduced transition metals were higher after high-voltage cycling (2.0–4.7 V versus Li/Li + ) than after lower-voltage cycling (2.0–4.3 V versus Li/Li + ). These results suggest that the layered lattice is disrupted at high voltages resulting in a formation of a metastable phase that is readily reduced under discharging conditions. Presumably, the surface reduced layer creates a passivation layer that inhibits efficient lithium diffusion, thus adversely impacting capacity retention. This hypothesis is further justified by several control experiments. First, after high-voltage cycling, the electrodes could not be revitalized to the initial state by reassembling the cell with fresh electrolytic solution ( Supplementary Fig. 15a ), because this did not reduce the impedance ( Fig. 2d ). Second, the capacity normally obtained with low-voltage cycling (2.0–4.3 V versus Li/Li + ) could not be restored after high-voltage cycling ( Supplementary Fig. 15b ). Third, the high-voltage capacity could be improved only by using an extremely slow charge–discharge rate even after 20 high-voltage cycles ( Supplementary Fig. 15c ). These observations indicate that the cycling losses imposed by high-voltage cycling are mainly due to the impedance rise caused by the surface reduced layer and SRL rather than changes in the bulk electrode material. 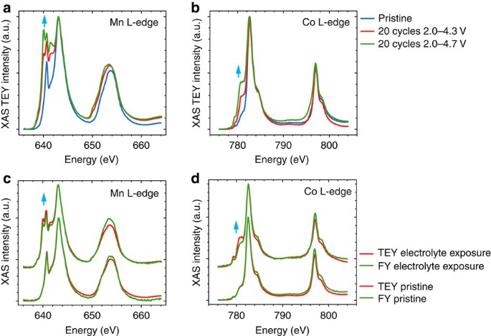Figure 4: Effects of cycling voltages and electrolyte exposure. (a) Mn L-edge XAS/TEY spectra and (b) Co L-edge XAS/TEY spectra of pristine and cycled electrodes (20 cycles). (c) Mn L-edge XAS/TEY/FY spectra and (d) Co L-edge XAS/TEY/FY spectra of a pristine electrode and one exposed to electrolytic solution for 7 days. The blue arrows in (a–d) indicate the increase of transition metals having low oxidation states. Figure 4: Effects of cycling voltages and electrolyte exposure. ( a ) Mn L-edge XAS/TEY spectra and ( b ) Co L-edge XAS/TEY spectra of pristine and cycled electrodes (20 cycles). ( c ) Mn L-edge XAS/TEY/FY spectra and ( d ) Co L-edge XAS/TEY/FY spectra of a pristine electrode and one exposed to electrolytic solution for 7 days. The blue arrows in ( a – d ) indicate the increase of transition metals having low oxidation states. Full size image Previous studies have attributed the surface reduced layer mainly to electrochemical processes with little attention dedicated to the effects of electrode–electrolyte reactivity [4] , [5] , [17] . Here we found that a surface reduced layer similar to the ones observed during high-voltage cycling is also created after an NMC electrode was immersed in the electrolyte ( Fig. 4c,d ), although it is thinner. In addition, its buildup leads to gradually increased charge transfer resistance ( Fig. 2e ). After extended cycling, the surface reduced layer originates from dual effects involving both the electrode–electrolyte reactivity and electrochemical activation. The immediate generation of the reduced surface upon exposure to electrolyte may also be responsible for the first-cycle coulombic inefficiencies that are usually observed with NMC electrodes even when cycled conservatively, using voltage limits well below the oxidative stability limit of the electrolytic solution. In the above discussion, XAS and EELS spectroscopies provided correlated evidence for the surface reduced layer and chemical evolution via the elucidation of local electronic structures primarily at the vicinity of NMC particle surfaces. The changes in electronic structures must be associated with the collapse and rearrangement of local crystal structures; that is, lattice reconstruction. The atomic resolution ADF-STEM imaging allows the visualization of the localized structural rearrangements at surfaces with the sensitivity of a single atom. A surface reconstruction layer is readily observed after the electrolyte exposure experiment ( Fig. 5a ), where the blue line indicates the boundary between the NMC layered structure and the surface reconstruction layer. This instantaneously generated reconstruction layer adversely impacts the capacity and first-cycle coulombic efficiency. The thickness of the surface reconstruction layer increased after one complete cycle between 2.0–4.7 V ( Fig. 5b ) relative to that observed on the particle that was exposed to the electrolytic solution without electrochemical cycling (although the duration of the two experiments was identical). The observation visually validates our previous conclusion that this layer originated from dual effects involving both electrode–electrolyte reactivity and electrochemical activation. The crystal structure of the reconstruction layer consists primarily of an rock-salt structure ( Fig. 5c,d ), with a few atomic layers of spinel structure as a ‘bridge’ between the layered structure (containing Ni 2+ , Mn 4+ and Co 3+ ) and rock-salt structure (containing Ni 2+ , Mn 2+ and Co 2+ ). By analysing a large number of ADF-STEM images, we found that the surface reconstruction layer was greatly influenced by crystal orientations. 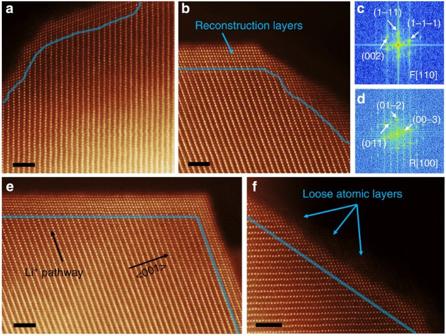Figure 5: Atomic resolution ADF-STEM images of NMC particles. (a) After electrolyte exposure (the exposure time is ~30 h, equivalent to the time used for one full cycle in this study). (b) After 1 cycle (2.0–4.7 V); the blue arrow indicates the surface reconstruction layer. (c,d) FFT results showing the surface reconstruction layer ([110] zone axis) and the NMC layered structure ([100] zone axis), respectively in (b). (e) Showing variation of the surface reconstruction layer thickness on orientation after 1 cycle (2.0–4.7 V). (f) Image showing loose atomic layers on an NMC particle, after 1 cycle (2.0–4.7 V). The blue lines indicate the boundaries between the NMC layered structure and surface reconstruction layer in all images. The scale bars are 2 nm in all images. Figure 5e shows a typical example of orientation-dependent surface reconstruction (more relevant images are available in Supplementary Fig. 16 ). Furthermore, reconstruction-poor and -rich surfaces are occasionally observed on the same NMC particle after cycling ( Supplementary Fig. 16 ). Due to the random orientation of NMC particles on the electrode surfaces, surface-sensitive XAS spectroscopy (that is, AEY, TEY) yields an average of the electronic structures for reconstruction-poor and -rich surfaces, and thus the high-energy components of XAS/AEY and XAS/TEY are still present in the electrodes that have been cycled ( Fig. 3c,d ). In general, the thicker surface reconstruction layers are observed along the lithium diffusion channels relative to other orientations (for example, 001 ), suggesting that surface reconstruction is promoted by lithium removal during charging, and the reconstruction is more severe in the regions that undergo dynamic lithium transport. Interestingly, we also observed dangling layers (that is, loose atomic layers) of the cubic rock-salt structure (indicated by blue arrows in Fig. 5f ) at the external surface of reconstruction layers. These loosely attached atomic layers are susceptible to dissolution into electrolytes and coincide with the suspected Mn 2+ dissolution in a variety of Mn-containing cathodes [42] , [43] , [44] . It has been shown in Supplementary Fig. 15c that, after 20 high-voltage cycles, the discharge capacity could be nearly recovered at a slow rate (190 mAh g −1 , compared with the first-cycle discharge capacity of 210 mAh g −1 ). Therefore, the transition metal dissolution accounts for a capacity loss of no more than 20 mAh g −1 . Figure 5: Atomic resolution ADF-STEM images of NMC particles. ( a ) After electrolyte exposure (the exposure time is ~30 h, equivalent to the time used for one full cycle in this study). ( b ) After 1 cycle (2.0–4.7 V); the blue arrow indicates the surface reconstruction layer. ( c , d ) FFT results showing the surface reconstruction layer ( [110] zone axis) and the NMC layered structure ( [100] zone axis), respectively in ( b ). ( e ) Showing variation of the surface reconstruction layer thickness on orientation after 1 cycle (2.0–4.7 V). ( f ) Image showing loose atomic layers on an NMC particle, after 1 cycle (2.0–4.7 V). The blue lines indicate the boundaries between the NMC layered structure and surface reconstruction layer in all images. The scale bars are 2 nm in all images. Full size image Finally, we performed density functional theory (DFT) calculation for the formation energy of the rock-salt structure from the layered structure as a function of lithium concentration ( Supplementary Fig. 17 ). Under oxygen partial pressure ranging from 10 −12 atm to 1 atm, we found that after about 60% of lithium has been removed from the NMC structure, it becomes favourable to form the rock-salt structure (that is, negative formation energy). This supports the above results showing that the high-voltage cycling (that is, more lithium ions are removed) leads to a much more severe buildup of the surface reduced layer (that is, rock-salt structure). Our experimental results showed that the to transition primarily occurred at the surface and direct exposure to electrolytic solution assisted the kinetics of this phase transition. We correlated cycling performance with the observation of structural reconstruction and chemical evolution at the surfaces of stoichiometric NMC materials using statistically viable high-throughput ensemble-averaged XAS as well as spatially resolved EELS and atomically resolved ADF-STEM imaging. The structural reconstruction was directly evidenced by the changes in the transition metal oxidation states and the atomic packing, which were achieved by synchrotron XAS and ADF-STEM, respectively. Our findings show that the challenge of achieving stable high-voltage cycling of the NMC electrodes lies with structural and chemical metastability at the surfaces. Upon cycling and/or electrolyte exposure, the surfaces of NMC particles undergo progressive reconstruction (that is, lower transition metal oxidation states, Fig. 3a,b ) from an –layered structure to an rock-salt structure in addition to the buildup of a complex SRL containing LiF and organic components (that is, chemical evolution). These observations provide new insights into the capacity degradation and impedance buildup in stoichiometric NMC materials undergoing high-voltage cycling conditions. Interestingly, the structural reconstruction at the surface is highly anisotropic, and primarily occurs along the lithium ion transport direction. This phenomenon would have been omitted without such a study at complementary length scales. This finding suggests that conformal protection coatings on certain orientations of NMC particles should be more beneficial than those on other orientations provided that the conformal coating is capable of inhibiting surface reconstruction and allows for efficient lithium diffusion. Preparation of electrode materials LiNi 0.4 Mn 0.4 Co 0.18 Ti 0.02 O 2 materials were synthesized using a co-precipitation method. For the synthesis of LiNi 0.4 Mn 0.4 Co 0.18 Ti 0.02 O 2 , 250 ml of an aqueous solution of transition metal nitrates (0.16 M Ni(NO 3 ) 2 , 0.16 M Mn(NO 3 ) 2 , 0.072 M Co(NO 3 ) 2 ), 0.008 M TiO(SO 4 )·xH 2 O and 250 ml of 0.8 M LiOH aqueous solution were dripped simultaneously into a beaker using a Masterflex C/L peristaltic pump and stirred continuously. The precipitate was collected, filtered and washed with DI water, and then dried overnight at 100 °C in the oven. The dried precipitate was ball-milled with LiOH or Li 2 CO 3 and then heated in air at 900 °C for 3 h with a ramp of 2 °C min −1 . The use of Li 2 CO 3 led to smaller NMC particles than that of LiOH. In the main text and Supplementary Information , the small and large NMC particles represent the materials made with Li 2 CO 3 and LiOH, respectively. Coin cell preparation and electrochemical measurements Composite electrodes were prepared with 84 wt% active material, 8 wt% polyvinylidene fluoride (Kureha Chemical), 4 wt% acetylene carbon black (Denka, 50% compressed) and 4 wt% SFG-6 synthetic graphite (Timcal, Graphites and Technologies) in N -methyl-2-pyrrolidinone and cast onto carbon-coated aluminium current collectors (Exopack Advanced Coatings ( http://www.exopackadvancedcoatings.com ) with typical active material loadings of 6–7 mg cm −2 . 2032 coin cells were assembled in a helium-filled glove box using the composite electrode as the positive electrode and Li metal as the negative electrode. A Celgard 2400 separator and 1 M LiPF 6 electrolyte solution in 1:2 w/w ethylene carbonate/dimethyl carbonate (Ferro Corporation) were used to fabricate the coin cells. Battery testing was performed on a computer controlled VMP3 potentiostat/galvanostat (BioLogic). 1C was defined as fully charging a cathode in 1 h, corresponding to a specific current density of 280 mA g −1 . Electrochemical impedance spectra were collected using a 10 mV AC signal ranging from 10 mHz to 100 kHz using this same instrument. The electrodes were removed from coin cells, rinsed with dimethyl carbonate and dried in a helium-filled glove box for further study. The electrodes were sealed under helium and then transferred to the synchrotron beamline using a homemade system to prevent air exposure. For electron microscopy and spectroscopy measurements, the electrode particles were scratched off and deposited onto TEM grids. Materials characterization X-ray diffraction (XRD) on powder samples was performed on a Bruker D2 Phaser diffractometer using CuKα radiation. Scanning electron microscopy (SEM) was performed on a JEOL JSM-7000F with a Thermo Scientific. EDS (energy dispersive X-ray spectroscopy) detector. XAS measurements were performed on the 31-pole wiggler beamline 10-1 at Stanford Synchrotron Radiation Lightsource using a ring current of 350 mA and a 1,000 l mm −1 spherical grating monochromator with 20 μm entrance and exit slits, providing ~1011, ph s −1 at 0.2 eV resolution in a 1 mm 2 beam spot. During the measurements, all battery electrode samples were attached to an aluminium sample holder using conductive carbon. Data were acquired under ultrahigh vacuum (10 −9 Torr) in a single load at room temperature using TEY, AEY and FY. The sample drain current was collected for TEY. AEY was collected with a Cylindrical Mirror Analyzer using pass energy of 200 eV and a kinetic energy window of 2 eV near the main Auger for oxygen and nitrogen, respectively. A silicon diode (IRD AXUV-100) was used to collect the FY positioned near the sample surface. Contributions from visible light were carefully minimized before the acquisition, and all spectra were normalized by the current from freshly evaporated gold on a fine grid positioned upstream of the main chamber. XAS signals were collected at several positions on individual electrodes to ensure that data were representative of the sample. A 200 keV and 300 keV probe-corrected field-emission scanning/transmission electron microscopes (S/TEM) were used for ADF-STEM imaging and spatially resolved EELS. Spectroscopic imaging was performed with an Enfina spectrometer on a Hitachi 2700C dedicated STEM. Calculation method The calculations were carried out using Kohn–Sham DFT with the projector augmented wave method, as implemented in the Vienna ab initio Simulation Package. For the exchange and correlation functional, we use a standard DFT+U framework with spin-dependent generalized gradient approximation of Perdew, Burke and Ernzerhof (PBE) [45] , [46] , [47] , [48] , [49] , [50] . The electron states were sampled using a k-point grid of 2 × 2 × 2 centred at the origin. The electronic wave functions were expanded in a plane wave basis set with an energy cutoff of 500 eV, and the ionic positions were optimized until the forces on the ions were converged to 10 meV/Å. The layered NMC material was modelled employing 27 unit cells with a superstructure with space group P3 1 12, while the rock-salt structured used space group employing the same configurational order for the cations as the NMC material. The generalized gradient approximation+U formalism developed by Dudarev et al . [51] was employed for the 3 d electrons of each transition metal cation species. The values of these Hubbard-U parameters for Ni, Mn and Co were initially determined from previous computational work on Li intercalation compounds [52] , and subsequently optimized by iteratively calculating the voltage profile as described by Meng and Dompablo [53] , to the values of 5.5 eV, 7.0 eV and 5.0 eV, respectively. In order to determine the relative stability of the layered versus rock-salt structure, the reaction free energy was calculated for the following reaction at different initial lithium concentrations. The Gibbs free energy for solid species were approximated by the zero temperature energies, neglecting vibrational contributions and assuming that the configurational disorder in the Ni, Co and Mn sublattice is frozen in at the temperatures of interest. For the oxygen molecule energy, the Gibbs free energy was computed using a standard ‘ ab initio thermodynamics’ formalism, in which the free energy is decomposed into three parts: (i) a zero temperature energy calculated from DFT, and corrected by an overbinding error as described in ref. 54 (ii) the zero-point energy of the oxygen molecule, (iii) finite temperature contributions arising from vibrational, translational and orientational motion, and taken from experimental measurements corresponding to a temperature of 298 K and a partial pressure of 1 atm [55] , and (iv) a term to account for variations of the oxygen partial pressure for 1 atm, 10 −6 atm and 10 −12 atm. How to cite this article : Lin, F. et al . Surface reconstruction and chemical evolution of stoichiometric layered cathode materials for lithium-ion batteries. Nat. Commun. 5:3529 doi: 10.1038/ncomms4529 (2014).